Emergent quantum confinement at topological insulator surfaces Topological insulators are an exotic state of quantum matter, guaranteed to have metallic edge or surface states due to an inverted ordering of their bulk electronic bands [1] . The corresponding topological invariants [2] dictate that there must be an odd number of such states intersecting the Fermi level between each pair of surface time-reversal invariant momenta. In the most widely investigated bismuth-chalchogenide family of topological insulators, there is just one of these so-called topological surface states (TSSs) creating a single Dirac cone around the Brillouin zone centre [3] , [4] , [5] , [6] . These materials are therefore widely regarded ideal templates to realize the predicted exotic phenomena and applications of this TSS. However, exposure to even the minute amount of residual gas in an ultra-high vacuum chamber induces a drastic reconstruction of the surface electronic structure. The Dirac point shifts to higher binding energies, indicating more electron-rich surfaces [7] , [8] , [9] , [10] . More importantly, additional pairs of two-dimensional, almost parabolic states emerge in the vicinity of the bulk conduction band [7] , which develop large Rashba-type splittings [8] , whereas new ladders of M-shaped states are created in the original bulk valence bands [7] , [11] . Given their propensity for formation, these must be considered part of the intrinsic electronic structure of the surface of any realistic topological insulator, for example when exposed to air or interfaced to another material. However, their existence is not predicted by idealized theoretical models of the bulk-truncated surface [3] , and has proved controversial. Recent proposals attribute their formation to a variety of electronic or structural modifications of the crystal host [7] , [8] , [9] , [11] , [12] , [13] , [14] , [15] , [16] , [17] , [18] , [19] , [20] , [21] , [22] , but to date no single model has been able to simultaneously reproduce the number and binding energies of the experimentally observed electronic states as well as the magnitude of their measured Rashba-type splittings. In the following, we show that this can be achieved taking account of only a single electronic phenomenon—a near-surface electrostatic potential variation. Such intrinsic electric fields are familiar from surface space-charge regions in conventional semiconductors [23] , [24] , and are also formed at interfaces where they can be modulated using applied gate voltages. Thus, our findings are not only relevant to understand the free surfaces of generic topological insulators, but also their use in transistor-style or other thin-film device architectures, which may ultimately provide one of the most promising routes towards spintronics. Our study elucidates the crucial interplay of quantum confinement with topological order for such systems, and uncovers a unique spin texture of the resulting electronic states. We consider Bi 2 Se 3 as a model example, but our computational approach can be freely adapted to virtually all topological insulators, such as other emerging Bi-chalcogenides or the half-Heusler alloys [25] , where we would expect a similarly striking role of band bending at free surfaces, interfaces, or in devices. Band-bending-driven quantum confinement We implement such a band bending scenario ( Fig. 1a ) within a 120 quintuple-layer tight-binding supercell calculation (see Methods ). Without incorporating any band bending, our supercell model yields a single TSS spanning from the bulk valence to conduction bands ( Supplementary Fig. S1 ), in good agreement with both first-principles slab calculations [3] and our experimental measurements of the pristine surface ( Supplementary Fig. S2 ). Additionally including an electrostatic potential variation, we find a hierarchy of electronic states emerges that is in excellent agreement with our experimental angle-resolved photoemission (ARPES) measurements of a doped topological insulator surface ( Fig. 1b ). The effective mass is slightly overestimated in our model, which stems from a small overestimation of this quantity in our bulk band structure calculations. Nonetheless, all other features are well reproduced. This agreement is remarkable, given that we do not adjust any parameters in our calculation. All tight-binding matrix elements are obtained from an ab initio calculation of the bulk electronic structure. The magnitude of the potential change is fixed by the experimentally measured shift of the Dirac point between a pristine-cleaved surface and the n -type doped one (see Supplementary Fig. S2 ), and its functional form follows from a solution of Poisson's equation [26] . 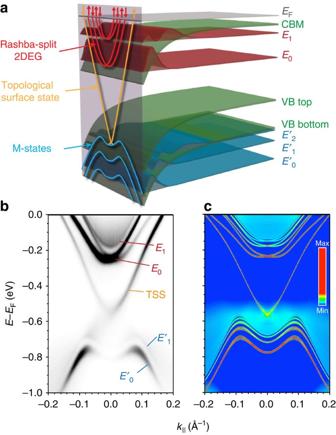Figure 1: Band-bending-induced surface electronic structure of Bi2Se3. (a) A near-surface electrostatic potential variation causes downward band bending of both the conduction band minimum (CBM) and valence band (VB) edges, forming a surface quantum well. It shifts the Dirac point of the TSS (yellow band) further below the Fermi level and causes the conduction band states to be restructured into ladders of Rashba-split two-dimensional subbands,En(red bands), with envelope wave functions (dark red) peaked close to the surface. A schematic spin texture of these states is shown by the arrows. The finite valence band width provides simultaneous confinement of the valence band states, causing these to also become quantized into ladders of M-shaped states,En′(blue bands). These features can all be seen in ARPES measurements of the surface electronic structure (b) and are well described by the surface projection (that is, real-space projection onto the first three quintuple layers) of anab initio-derived tight-binding model (c) of the ideal Bi2Se3bulk structure subject only to a perturbing electrostatic potential close to the surface (false colour scale inset).k|is along the Γ–M direction. Figure 1: Band-bending-induced surface electronic structure of Bi 2 Se 3 . ( a ) A near-surface electrostatic potential variation causes downward band bending of both the conduction band minimum (CBM) and valence band (VB) edges, forming a surface quantum well. It shifts the Dirac point of the TSS (yellow band) further below the Fermi level and causes the conduction band states to be restructured into ladders of Rashba-split two-dimensional subbands, E n (red bands), with envelope wave functions (dark red) peaked close to the surface. A schematic spin texture of these states is shown by the arrows. The finite valence band width provides simultaneous confinement of the valence band states, causing these to also become quantized into ladders of M-shaped states, E n ′(blue bands). These features can all be seen in ARPES measurements of the surface electronic structure ( b ) and are well described by the surface projection (that is, real-space projection onto the first three quintuple layers) of an ab initio -derived tight-binding model ( c ) of the ideal Bi 2 Se 3 bulk structure subject only to a perturbing electrostatic potential close to the surface (false colour scale inset). k | is along the Γ–M direction. Full size image All of the new electronic states observed experimentally arise simply due to the perturbative effect of this electrostatic potential in the system, which causes a triangular-like downward bending of the bulk electronic bands close to the surface by almost 250 meV ( Fig. 2b ). Combined with the large potential step at the material/vacuum interface, this creates a near-surface quantum well for electrons. The bulk conduction band states are consequently restructured into ladders of multiple subband states [7] , [27] , [28] . Our layer-resolved calculations ( Fig. 2 ) show that the lowest such subband, lying deep within the potential well, is localized in the topmost few quintuple layers of the structure: The electrons that populate this subband are free to move parallel to the surface, but are strongly confined perpendicular to it, forming a two-dimensional electron gas (2DEG). This state exhibits a strong Rashba spin–orbit splitting, whose calculated magnitude reproduces our experimental observations. Higher-lying states of the subband ladder are less strongly bound within the surface quantum well and contribute significant weight as far as 10–15 quintuple layers below the sample surface. The smaller spin splitting observed experimentally for these higher-lying states is again reproduced by our model calculations, confirming that the Rashba splitting is driven by the potential gradient of the confining electrostatic potential [8] . Similar to the conduction band 2DEG, a ladder of subbands is also observed in the valence band near the zone centre. These hole-like states become quantum confined between the surface and the upper edge of a projected bulk band gap [3] , [11] , as shown schematically in Fig. 1a . The lowest of these, as for the topological and lower conduction-band quantum well states, is strongly confined within the first 3–4 quintuple layers below the surface. We also find a small spin splitting of these valence band quantum well states, which is not resolved experimentally. Its location, around the top of their M-shaped dispersions, indicates a subtle interplay of spin–orbit interactions between the valence and conduction band subbands [29] . Thus, a hierarchy of electronic states in both energy and spatial extent is created, spanning from the two-dimensional limit of the TSS and lowest subbands of the conduction and valence bands to the three-dimensional continuum ( Fig. 1a ). 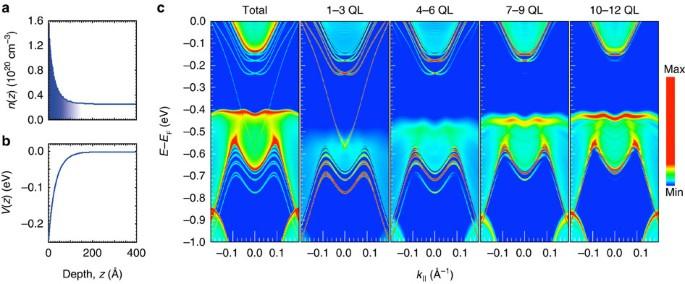Figure 2: Confinement of the electronic states. (a,b) show the depth-dependence of the carrier density,n(z), and potential profile,V(z), near the surface of Bi2Se3, respectively. The blue shading schematically represents the spatial extent of the surface-localized 2DEG. (c) Quintuple-layer (QL) projected supercell calculations of the electronic structure along Γ–M, revealing the varying spatial confinement of the different electronic states (false colour scale shown to right). Figure 2: Confinement of the electronic states. ( a , b ) show the depth-dependence of the carrier density, n ( z ), and potential profile, V ( z ), near the surface of Bi 2 Se 3 , respectively. The blue shading schematically represents the spatial extent of the surface-localized 2DEG. ( c ) Quintuple-layer (QL) projected supercell calculations of the electronic structure along Γ–M, revealing the varying spatial confinement of the different electronic states (false colour scale shown to right). Full size image Three-dimensional spin texture Intriguingly, we find an anticorrelation between this electronic dimensionality, and that of the states' spin texture. This is revealed experimentally via an asymmetry in the matrix element for photoemission when the system is excited by right and left circularly polarized light, respectively ( Fig. 3a–c ). Such circular dichroism has previously been suggested to probe the spin of the isolated TSS, although the microscopic origin of the dichroism has proved controversial [30] , [31] , [32] , [33] , [34] . Recently, Park et al . [31] proposed the existence of an unquenched local orbital angular momentum (OAM) of the TSS. They found that this has the same chiral structure as the spin angular momentum (SAM), permitting the well known spin-momentum locking of the TSS, but opposite helicity due to the strong spin–orbit coupling. They proposed that the observed dichroism in ARPES measurements of the TSS results due to this orbital texture. Such circular dichroism, therefore, still reveals the spin texture of the system (up to an arbitrary sign), but indirectly via the orbital sector. We therefore employ this to extract the relative spin texture of the entire low-energy electronic structure of the surfaces of topological insulators. We note that, for the relative changes in dichroism between the bands that we study here we can neglect final-state effects, as transitions from all of these closely spaced initial states will go into the same (broad) final state. 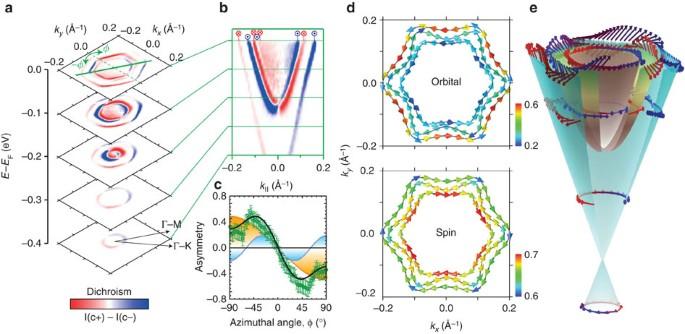Figure 3: Three-dimensional orbital and spin texture of the topological and 2DEG states. (a,b) Circular dichroism in constant energy contours andEversuskdispersions measured by ARPES encode the spin–orbital texture of the topological (outer band) and 2DEG (remaining features) states. Circular dichroism along Γ–M (b), extracted along the bold green line shown ina, contains only the in-plane component. This reveals opposite helicity for consecutive Fermi surface sheets, with the spin pointing into () or out of () the plane of the figure. (c) Quantitative analysis of the angular dependence of the dichroism around the Fermi surface, shown for the outer branch of the lowest Rashba-split 2DEG state as a function of aziumthal angle,φ, from the dashed green line (Γ–M,ky=0) direction shown ina. Error bars reflect an approximate estimate of the uncertainty in extracting the asymmetry parameter from the experimental measurements, incorporating statistical errors in peak fitting, systematic errors and sample-to-sample variations. The fit to the total dichroism (black line) contains not only a component which varies as sin(φ) (yellow), but also a large sin(3φ) contribution (blue), revealing a significant out-of-plane orbital, and therefore also spin, canting. This is consistent with our calculations shown ind(see alsoSupplementary Fig. S5), which reveal an alternating helical texture of both the orbital and spin angular momenta (absolute magnitude represented by the false colour scale to the right), but with opposite winding direction. These develop significant out-of-plane components for the larger Fermi surface sheets. In contrast, our calculations and experiment reveal that all other states largely retain the in-plane spin texture characteristic of classic Rashba systems all the way up to the Fermi energy. Together, this leads to a rich three-dimensional spin-texture of the surface electronic structure of topological insulators, as summarized by the arrows on the TSS (blue) and lowest Rashba-split (brown-green) subband of the 2DEG ine. Figure 3: Three-dimensional orbital and spin texture of the topological and 2DEG states. ( a , b ) Circular dichroism in constant energy contours and E versus k dispersions measured by ARPES encode the spin–orbital texture of the topological (outer band) and 2DEG (remaining features) states. Circular dichroism along Γ–M ( b ), extracted along the bold green line shown in a , contains only the in-plane component. This reveals opposite helicity for consecutive Fermi surface sheets, with the spin pointing into ( ) or out of ( ) the plane of the figure. ( c ) Quantitative analysis of the angular dependence of the dichroism around the Fermi surface, shown for the outer branch of the lowest Rashba-split 2DEG state as a function of aziumthal angle, φ , from the dashed green line (Γ–M, k y =0) direction shown in a . Error bars reflect an approximate estimate of the uncertainty in extracting the asymmetry parameter from the experimental measurements, incorporating statistical errors in peak fitting, systematic errors and sample-to-sample variations. The fit to the total dichroism (black line) contains not only a component which varies as sin( φ ) (yellow), but also a large sin(3 φ ) contribution (blue), revealing a significant out-of-plane orbital, and therefore also spin, canting. This is consistent with our calculations shown in d (see also Supplementary Fig. S5 ), which reveal an alternating helical texture of both the orbital and spin angular momenta (absolute magnitude represented by the false colour scale to the right), but with opposite winding direction. These develop significant out-of-plane components for the larger Fermi surface sheets. In contrast, our calculations and experiment reveal that all other states largely retain the in-plane spin texture characteristic of classic Rashba systems all the way up to the Fermi energy. Together, this leads to a rich three-dimensional spin-texture of the surface electronic structure of topological insulators, as summarized by the arrows on the TSS (blue) and lowest Rashba-split (brown-green) subband of the 2DEG in e . Full size image Along the Γ–M mirror direction, symmetry requires that the spin, and therefore also the OAM, must lie entirely within the surface plane [35] . Our measurements of circular dichroism extracted along this direction ( Fig. 1b ) are therefore representative of the in-plane spin–orbital texture. The dichroism changes sign upon moving inwards from the outermost Fermi surface sheet of the topological state to the subsequent Fermi surfaces of the lowest Rashba-split subband ( E 0 ) of the 2DEG. This is entirely consistent with the results of spin-resolved photoemission for these states [8] . More extensive analysis ( Supplementary Fig. S3 ) indicates that this trend continues for the next 2DEG subband. Given the left-handed helicity of the TSS [9] , these measurements therefore indicate an alternating left–right–left–right–left helicity for the spin of consecutive Fermi surface sheets of the TSS and first ( E 0 ) and second ( E 1 ) quantized conduction subbands. Away from this direction, dichroism of the inner E 0 and E 1 2DEG Fermi surface sheets vary sinusoidally with angle, φ , around the Fermi surface (shown in Supplementary Fig. S3 ). This reveals a model Rashba-like [36] helical spin texture of these states, with the spin-polarized entirely in the surface plane at all energies. However, for the more spatially localized TSS and outermost 2DEG state, the dichroism additionally develops a strong sin(3 φ ) component, which is maximal along Γ–K and zero along Γ–M ( Fig. 1c and Supplementary Fig. S3 ). This reflects a strong out-of-plane spin polarization close to the Fermi level, which is correlated with hexagonal warping of the electronic states [35] , [36] , [37] , [38] , [39] , again switches sign between neighbouring states, and decreases with increasing binding energy ( Supplementary Fig. S4 ). These findings are fully supported by our tight-binding supercell calculations ( Fig. 3d ; Supplementary Fig. S5 ), where we find that the OAM and SAM exhibit an alternating helical structure for consecutive Fermi surface sheets, both also developing increasing out-of-plane components with hexagonal warping. The local OAM, therefore, similar to the spin texture, does lie purely in the surface plane at k -points along Γ–M, whereas away from this high-symmetry direction it gradually attains a net out-of-plane component, which is maximal along Γ–K. However, the OAM helicity of each band is opposite to that of its SAM. This not only confirms that the TSS possesses intricately related OAM and SAM structures, but also reveals that the non-trivial topology drives the TSS and 2DEG states to have a novel alternating helical OAM texture. Thus, not only does the band bending promote the creation of additional Fermi surface sheets, it also leads to complex band- and binding-energy-dependent three-dimensional orbital- and spin textures of the resulting electronic system, as summarized for the spin in Fig. 3e . Together, this will cause significant complications for the interpretation of spin-dependent transport experiments, and inter-band processes will weaken the topological protection against backscattering commonly assumed for the TSS of these compounds. Nonetheless, we note that our resolution limited linewidths of full width at half maximum indicate that the intrinsic scattering remains relatively weak for all Fermi surface sheets. Surface-bulk connectivity The complex spin texture of these states also raises questions over their interplay. For any system with time-reversal symmetry, the electronic states must be spin-degenerate at time-reversal invariant momenta, even though a breaking of inversion symmetry by the confining potential and surface allows a lifting of the spin degeneracy at arbitrary k -points. The hexagonal Brillouin zone of the Bi 2 Se 3 surface contains time-reversal invariant k -points at the zone centre (Γ point) and at the side-centre (M) point. 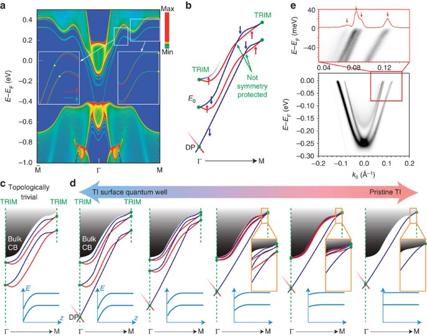Figure 4: Connectivity of the surface electronic spectrum. (a) Full electronic structure calculation along the Γ–M direction. At the Γ point, Kramer's degeneracy requires that the TSS is spin-degenerate (the Dirac point, DP) and each 2DEG state is degenerate with its spin-split pair. At the M-point, this degeneracy occurs between the topological state and outer branch of the lowest 2DEG state, and then between the inner and outer branch of each successive pair of 2DEG states, as shown schematically inb. This forces a divergence of the spin-up (red, up arrows) and spin-down (blue, down arrows) branches of each subband at high wavevectors, in contrast to topologically trivial Rashba systems (c). (d) Schematic evolution of the band connectivity to the bulk of topological insulators as a function of surface band bending (inset), with degeneracy between spin-up (red) and spin-down (blue) bands always maintained at the Γ and M points. Between these time-reversal invariant momenta (TRIM), no fundamental symmetry dictates degeneracy of the states. Although additional accidental degeneracies can occur (a,b), our high-resolution ARPES measurements (e) reveal that, away from the zone centre, all bands remain nondegenerate up until at least the Fermi level. This is clearly observed in a magnified view near the Fermi level (red region), where four distinct peaks arising from spin-split 2DEG states (identified by small arrows) can be resolved in the Fermi level momentum distribution curve. Figure 4a shows the electronic structure calculated along the entire Γ–M direction. At the Γ point, each Rashba-split pair of 2DEG states clearly become degenerate. For the TSS, this initially appears to be complicated by the presence of bulk states, with the Dirac point looking to be buried deep in the bulk valence band. However, locally, the TSS is still situated within a projected band gap of the (bent) bulk bands, and so remains a well-defined surface state (unlike the 2DEG states that are located within, and indeed derived from, the projected bulk-like bands). Our layer-projected calculations ( Fig. 2 ) show that the Kramer's degeneracy of the TSS is preserved in the presence of the band-bending potential, contrary to previous suggestions of a band gap opening in the surface spectrum at the Dirac point [13] , [17] . Figure 4: Connectivity of the surface electronic spectrum. ( a ) Full electronic structure calculation along the Γ–M direction. At the Γ point, Kramer's degeneracy requires that the TSS is spin-degenerate (the Dirac point, DP) and each 2DEG state is degenerate with its spin-split pair. At the M-point, this degeneracy occurs between the topological state and outer branch of the lowest 2DEG state, and then between the inner and outer branch of each successive pair of 2DEG states, as shown schematically in b . This forces a divergence of the spin-up (red, up arrows) and spin-down (blue, down arrows) branches of each subband at high wavevectors, in contrast to topologically trivial Rashba systems ( c ). ( d ) Schematic evolution of the band connectivity to the bulk of topological insulators as a function of surface band bending (inset), with degeneracy between spin-up (red) and spin-down (blue) bands always maintained at the Γ and M points. Between these time-reversal invariant momenta (TRIM), no fundamental symmetry dictates degeneracy of the states. Although additional accidental degeneracies can occur ( a , b ), our high-resolution ARPES measurements ( e ) reveal that, away from the zone centre, all bands remain nondegenerate up until at least the Fermi level. This is clearly observed in a magnified view near the Fermi level (red region), where four distinct peaks arising from spin-split 2DEG states (identified by small arrows) can be resolved in the Fermi level momentum distribution curve. Full size image At the M-point, our calculations reveal that the TSS connects to the outer branch of the lower 2DEG state. Assuming a spin-down state for the TSS, the pairing 2DEG state has no other choice but to be spin-up. Its spin-down partner must then become connected with the outer branch of the second subband to satisfy TR symmetry for these states, thereby dictating the overall up–down–up–down–up spin configuration discussed above. Fundamentally, this pair-exchange follows from the non-trivial Z 2 topology of the bulk band structure. This requires that the TSS must connect from the bulk valence to conduction bands. Now, however, the original bulk bands have become quantized into two-dimensional subband states in the vicinity of the surface, and our calculations indicate that it is to these subbands which the topological state connects. If the band bending is reduced ( Fig. 4d ), the subband states will become split-off less far below the bulk conduction bands, while their Rashba spin splitting will simultaneously decrease. This will consequently reduce the relative energy separation of the multiple band connectivities at the M-point. Extending this continuously to the limit of no band bending, the subbands evolve into the lower bulk conduction band states, while the zone-edge connectivities merge into a single degeneracy at the M-point between the topological state and the bulk electronic continuum. This clarifies how the surface-bulk connectivity occurs in the idealized case of topological insulators with a pristine surface and no band bending. In the more realistic case where band bending is present, however, the surface-bulk connectivity is mediated via the quantum-well states. This requires the outer and inner branches of the spin–split subbands to diverge from each other at large k -vectors, in stark contrast to conventional Rashba systems [41] in which the two spin channels merge again at zone-edge time-reversal invariant momenta ( Fig. 4c ). In topologically trivial surface systems where giant Rashba effects have been observed, the spin splitting depends sensitively on details of the near-surface atomic coordinates relative to the surface potential step [42] . In contrast, because of the subband connectivity, the magnitude of the Rashba splitting in a topological insulator 2DEG is directly linked to the subband separation. The possibility to control the 2DEG spin splitting electrostatically via the band bending is therefore intrinsic to topological insulator 2DEGs, rendering these systems ideal candidates for applications in spintronics. Hexagonal warping of the electronic states can additionally induce accidental degeneracies along high-symmetry lines [43] , [44] , as seen in Fig. 4 . However, as these are not protected by any fundamental symmetry, introduction of perturbations in the system can shift, or even completely remove, such accidental degeneracies. Experimentally, the inner branch of the lower 2DEG state and outer branch of the upper 2DEG state can be seen to approach each other at low binding energies ( Fig. 4d ), consistent with their proximity to the accidental crossing predicted in our calculations. However, contrary to previous reports [13] , [17] , our high-resolution measurements reveal that the occupied bands remain nondegenerate and exhibit rather parallel dispersion close to the Fermi level, which could be indicative of an avoided crossing. The electronic structure that we consider here represents the generic surface electronic structure of topological insulators under realistic conditions, such as exposure to atmosphere [12] , [21] , or in desired devices such as the (spin-)transistor [8] . We have shown that this entire surface electronic system can be accurately described, considering only a single modification of the pristine crystal—a near-surface electrostatic potential variation. The quantitative agreement of our parameter-free tight-binding supercell calculations to our photoemission measurements demonstrates that such a band bending alone is sufficient to induce the entire experimentally measured complex electronic structure of topological insulator surfaces. We stress that our approach does not require any additional modifications beyond an electrostatic potential, such as a huge increased van der Waals gap size [15] , [16] , [18] , [20] , intercalation [45] , other artificial detachments of a finite number of crystal layers [14] , or the formation of new TSSs [13] . Despite its conceptual simplicity, the band bending has dramatic consequences for the surface electronic structure. Driven by an emergent role of quantum size effects, it leads to a rich surface electronic system simultaneously comprising both electron- and hole-like subbands of varying spatial confinement and with intertwined three-dimensional spin textures. We have shown how these subbands mediate connectivity of the bulk bands and the TSS, one of the defining properties of topological insulators, through a series of band degeneracies required by time-reversal symmetry, and further identify possible accidental degeneracies, which we do not observe experimentally. Understanding whether interactions not included in our theoretical treatment have a role in avoiding such accidental degeneracies will be crucial to unravel surface-bulk coupling in these materials, and the role of interactions in limiting mobilities of spin-polarized surface transport in topological insulators. Theory Relativistic electronic structure calculations were carried out within the context of density functional theory using the Perdew–Burke–Ernzerhof exchange-correlation functional [46] and the augmented plane wave plus atomic orbitals method as implemented in the WIEN2K program [47] . For all the atoms, the muffin-tin radius R MT was set to 2.5 Bohr and the maximum modulus of reciprocal vectors K max was chosen such that R MT K max =7.0. The primitive cell was considered to be hexagonal (space group: ) with lattice parameters and atomic positions taken from experiment [48] . The corresponding Brillouin zone was sampled using a 10 × 10 × 3 k -mesh. To simulate the effect of band bending, a 120 qunituple-layer tight-binding supercell Hamiltonian was constructed by downfolding the augmented plane wave plus atomic orbitals Hamiltonian using maximally localized Wannier functions [49] , [50] , [51] . We chose valence p orbitals of Bi and Se as the projection centres of the Wannier functions. The bending potential was obtained by solving the coupled Poisson–Schrödinger equation [26] , assuming a static dielectric constant of 70 (ref. 8 ). The resulting potential was then added to the onsite terms of the tight-binding supercell Hamiltonain. The (quintuple-layer-projected) surface band structure was eventually obtained by diagonalizing the supercell Hamiltonian (and projecting the resulting eigenstates onto the maximally localized Wannier functions of respective surface quintuple layers). Experiment Bi 2 Se 3 crystals were prepared by reacting high-purity elements (5 N) of Bi and Se in sealed, evacuated quartz tubes at 850 °C for 2 days, followed by cooling at 2–3 °C h −1 to 650 °C. The crystals were annealed at this temperature for 7 days before quenching to room temperature. ARPES measurements were performed at 10 K using circularly polarized light with photon energies of 20–30 eV and a Scienta R4000 hemispherical analyser at the SIS beamline of the Swiss Light Source. Surface doping was achieved by depositing potassium at room temperature on freshly cleaved samples from a properly outgassed SAES K getter source. The sample was then immediately transferred to the low-temperature manipulator for ARPES measurements. How to cite this article: Bahramy, M.S. et al . Emergent quantum confinement at topological insulator surfaces. Nat. Commun. 3:1159 doi: 10.1038/ncomms2162 (2012).